Aβ alters the connectivity of olfactory neurons in the absence of amyloid plaquesin vivo The amyloid beta peptide aggregates into amyloid plaques at presymptomatic stages of Alzheimer's disease, but the temporal relationship between plaque formation and neuronal dysfunction is poorly understood. Here we demonstrate that the connectivity of the peripheral olfactory neural circuit is perturbed in mice overexpressing human APPsw (Swedish mutation) before the onset of plaques. Expression of human APPsw exclusively in olfactory sensory neurons also perturbs connectivity with associated reductions in odour-evoked gene expression and olfactory acuity. By contrast, olfactory sensory neuron axons project correctly in mice overexpressing wild-type human amyloid precursor protein throughout the brain and in mice overexpressing M671V human APP, a missense mutation that reduces amyloid beta production, exclusively in olfactory sensory neurons. Furthermore, expression of Aβ40 or Aβ42 solely in the olfactory epithelium disrupts the olfactory sensory neuron axon targeting. Our data indicate that altering the structural connectivity and function of highly plastic neural circuits is one of the pleiotropic actions of soluble human amyloid beta. The pathobiology of Alzheimer's disease (AD) erodes neural networks and their underlying neural circuits, resulting in cognitive deficits and, ultimately, dementia [1] . Accumulations of amyloid beta (Aβ) peptide assemblies in the cortex, especially amyloid plaques, are present years before the onset of clinical symptoms of AD [2] . In fact, approximately 30% of cognitively intact septuagenarians harbour cerebral amyloid plaques [3] , [4] . Defining the temporal relationship between neural network dysfunction and amyloid deposition is crucial in developing effective therapies for the preclinical stage of AD [5] . Transgenic mice overexpressing pathogenic mutated alleles of the human amyloid precursor protein (hAPP) model the cerebral amyloidosis of preclinical AD [6] . In these models, neurons surrounding amyloid plaques exhibit reduced dendritic spine density and elevated resting intracellular calcium concentrations [7] , [8] . However, loss of synaptic proteins precede amyloid deposition in these models [9] and soluble Aβ species disrupt neural network function, for example, inhibiting long-term potentiation, inducing long-term depression and diminishing the density of dendritic spines [10] , [11] . Lentiviral expression of hAPP, but not M671V hAPP (hAPPmv; M671V, a synthetic missense mutation of hAPP, which impairs Aβ generation [12] ), in hippocampal slice preparations evoked a long-term depression-like phenotype and reduced spine density in adjacent neurons not expressing hAPP [13] , [14] , [15] . Together, these data indicate that soluble Aβ species, either released from cells or diffusing from the periphery of amyloid deposits, mediate neural circuit dysfunction. In this study, we probe the actions of human Aβ in the mouse peripheral olfactory neural circuit in vivo , a genetically tractable established model of neuronal connectivity. Interestingly, the neural network underpinning olfactory perception and odour naming is compromised early in AD [16] . Each mouse olfactory sensory neuron (OSN) expresses a single olfactory receptor (OR), choosing from over 1,000 OR genes [17] . Each OR gene can be modified to express marker proteins or disease genes in a defined OSN cell type with exquisite specificity. To a first approximation, this circuit is organized as over 1,000 parallel channels defined by OR proteins, which govern the response properties to odours [18] and the sites of axon projection on the surface of the olfactory bulb [19] , [20] . Collectively, these OR-dictated projection loci form a stereotyped map. We find that overexpression of the Swedish mutation of hAPP (hAPPsw), which causes early onset AD [21] , disrupts the connectivity of OSNs, reduces activity-dependent gene expression in second-order olfactory neurons and compromises olfactory acuity. These findings are not present in control mouse lines that overexpress wild-type hAPP or hAPPmv. Moreover, expression of Aβ40 or Aβ42 restricted to the olfactory epithelium also disturbs OSN axon targeting. These results indicate that human Aβ induces axon dysfunction in vivo in the absence of amyloid plaques. OSN axons mistarget in mice overexpressing hAPPsw Axons of OSNs expressing the same OR innervate discrete glomeruli on the surface of the olfactory bulb ( Fig. 1a ). The naturally occurring hAPPsw (K670N, M671L) augments cleavage by the β-secretase, thereby increasing Aβ production ( Fig. 1b ) [22] . We bred Tg2576 mice [22] , which overexpress hAPPsw throughout the brain, including OSNs in the olfactory epithelium ( Supplementary Fig. S1 ), with a mouse line in which the P2 OR gene was modified to also express green fluorescent protein (GFP) [20] . In control animals, a single glomerulus predominantly received fluorescent fibres in each bulb hemisphere. ( Fig. 1c,d ). By contrast, in littermate animals overexpressing hAPPsw, P2 axon projections terminate within multiple glomeruli per half bulb ( Fig. 1e,f ). 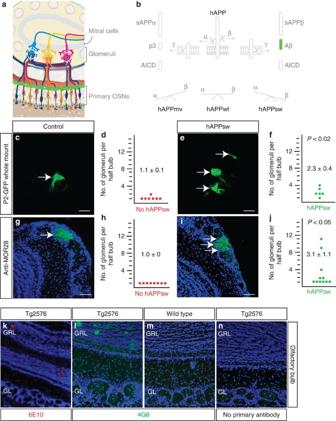Figure 1: Aberrant OSN projections in transgenic mouse lines overexpressing hAPPsw. (a) Schematic representation of the anatomy of the peripheral olfactory neural circuit demonstrating that choice of olfactory receptor (OR) (depicted by colour) dictates the projection target of its axon in the olfactory bulb. (b) Schematic representation of the protease cleavage pathways to generate Aβ and other fragments from hAPP. The mutation hAPPsw enhances flux through the β-secretase pathway, and M671V hAPP (hAPPmv) impairs flux through the β-secretase pathway. (c,d) Representative image of olfactory bulbs from P2-ires-GFP mice reveal a single glomerulus (indicated by arrow) per half bulb is targeted by axons containing GFP (each dot represents result per half bulb). (e,f) Representative image and quantification of olfactory bulbs from Tg2576 (panneuronal hAPPsw)/P2-ires-GFP mice reveal aberrant targeting of fibres containing GFP to multiple glomeruli (arrows) per half bulb (P<0.02, two-tailed Student'st-test;n=7 (controls);n=6 (Tg2576)). (g,h) Representative coronal section and quantification of olfactory bulbs from wild-type mice immunostained with anti-MOR28 and TOTO-3 reveal targeting to a single glomerulus (arrow). (i,j) Representative coronal section and quantification of olfactory bulbs from Tg2576 hAPPsw mice immunostained with anti-MOR28 and TOTO-3 reveal aberrant targeting of MOR28 axons to multiple glomeruli (arrows;P<0.05, two-tailed Student'st-test;n=8 (controls);n=11 (Tg2576)). Data presented as means±s.e.m. (k) The olfactory bulb from a 13-month-old Tg2576 mouse immunostained with 6E10 anti-APP antibody shows the presence of plaques in the granule cell layer (GRL). No plaques are seen in the glomerular layer (GL). (l–n) The human-specific antibody 4G8 reveals expression of hAPPsw in the glomerular layer (GL) of Tg2576 (24 months old), but not in wild-type mice (m) or when 4G8 is omitted from the Tg2576 tissue (n). Plaques are seen in GRL but not in the GL cell layers in the 24-month-old Tg2576 mouse (l). Scale bar=100 μm. Figure 1: Aberrant OSN projections in transgenic mouse lines overexpressing hAPPsw. ( a ) Schematic representation of the anatomy of the peripheral olfactory neural circuit demonstrating that choice of olfactory receptor (OR) (depicted by colour) dictates the projection target of its axon in the olfactory bulb. ( b ) Schematic representation of the protease cleavage pathways to generate Aβ and other fragments from hAPP. The mutation hAPPsw enhances flux through the β-secretase pathway, and M671V hAPP (hAPPmv) impairs flux through the β-secretase pathway. ( c,d ) Representative image of olfactory bulbs from P2-ires-GFP mice reveal a single glomerulus (indicated by arrow) per half bulb is targeted by axons containing GFP (each dot represents result per half bulb). ( e,f ) Representative image and quantification of olfactory bulbs from Tg2576 (panneuronal hAPPsw)/P2-ires-GFP mice reveal aberrant targeting of fibres containing GFP to multiple glomeruli (arrows) per half bulb ( P <0.02, two-tailed Student's t -test; n =7 (controls); n =6 (Tg2576)). ( g,h ) Representative coronal section and quantification of olfactory bulbs from wild-type mice immunostained with anti-MOR28 and TOTO-3 reveal targeting to a single glomerulus (arrow). ( i,j ) Representative coronal section and quantification of olfactory bulbs from Tg2576 hAPPsw mice immunostained with anti-MOR28 and TOTO-3 reveal aberrant targeting of MOR28 axons to multiple glomeruli (arrows; P <0.05, two-tailed Student's t -test; n =8 (controls); n =11 (Tg2576)). Data presented as means±s.e.m. ( k ) The olfactory bulb from a 13-month-old Tg2576 mouse immunostained with 6E10 anti-APP antibody shows the presence of plaques in the granule cell layer (GRL). No plaques are seen in the glomerular layer (GL). ( l–n ) The human-specific antibody 4G8 reveals expression of hAPPsw in the glomerular layer (GL) of Tg2576 (24 months old), but not in wild-type mice ( m ) or when 4G8 is omitted from the Tg2576 tissue ( n ). Plaques are seen in GRL but not in the GL cell layers in the 24-month-old Tg2576 mouse ( l ). Scale bar=100 μm. Full size image To confirm this phenotype, we examined a distinct subpopulation of OSNs expressing a different OR, MOR28. In control mice, axons labelled with an antibody against MOR28 [23] projected to only one glomerulus per half bulb ( Fig. 1g,h ). However, in Tg2576 mice, multiple adjacent glomeruli per half olfactory bulb received MOR28-labelled fibres ( Fig. 1i,j ). This phenotype was observed in both males and females, and at ages ranging from 10 days to 12 months. Thus, mistargeting of axons in the olfactory system occurs before plaque deposition in the olfactory bulbs of Tg2576 mice ( Fig. 1k–n ). Intact targeting in mice overexpressing wild-type hAPP In I5 mice overexpressing the wild-type hAPP gene ( hAPPwt ) [9] , immunostaining of the olfactory epithelium revealed robust expression of hAPPwt in OSNs ( Fig. 2a,b ). We bred the I5 mouse line with a line in which the P2 OR gene was modified to also express the fusion protein mouse tau-β-galactoside (tau-LacZ) [20] . Immunostaining of the olfactory bulb using an anti-LacZ antibody did not reveal differences in targeting of axons of OSNs expressing P2 ( Fig. 2c,d ). Similiarly, the fidelity of targeting of axons of OSNs expressing MOR28 was also preserved ( Fig. 2e,f ) relative to littermate controls. These preserved axon projection patterns suggest that overexpression of the hAPPsw allele alters connectivity of this neural circuit. 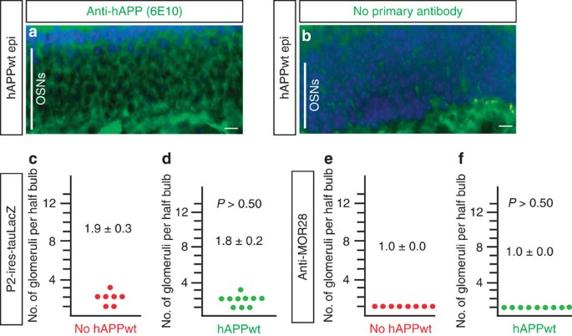Figure 2: Preserved OSN projections in transgenic mouse lines overexpressing hAPPwt. (a,b) Olfactory epithelia harvested from 12-week-old mice overexpressing the hAPP protein driven by the platelet-derived growth factor (PDGF) β-promotor expressed APP as shown by immunostaining with anti-APP 6E10 (a) relative to a no primary antibody control (b). Scale bar=20 μm. (c,d) Quantification of olfactory bulbs from control 1-year-old P2-ires-GFP mice and from I5 human wild-type APP (hAPPwt)-overexpressing mice reveal targeting of fibres containing GFP to two glomeruli per half bulb in both lines (P> 0.50, two-tailed Student'st-test;n=7 (controls);n=10 (I5)). (e,f) Quantification of olfactory bulbs from control mice and from I5 hAPPwt transgenic mice immunostained with anti-MOR28 reveal targeting to a single glomerulus (P>0.50, two-tailed Student'st-test;n=8 (controls);n=9 (I5)). Scale bar=100 μm. Data presented as means±s.e.m. Figure 2: Preserved OSN projections in transgenic mouse lines overexpressing hAPPwt. ( a,b ) Olfactory epithelia harvested from 12-week-old mice overexpressing the hAPP protein driven by the platelet-derived growth factor (PDGF) β-promotor expressed APP as shown by immunostaining with anti-APP 6E10 ( a ) relative to a no primary antibody control ( b ). Scale bar=20 μm. ( c,d ) Quantification of olfactory bulbs from control 1-year-old P2-ires-GFP mice and from I5 human wild-type APP (hAPPwt)-overexpressing mice reveal targeting of fibres containing GFP to two glomeruli per half bulb in both lines ( P > 0.50, two-tailed Student's t -test; n =7 (controls); n =10 (I5)). ( e,f ) Quantification of olfactory bulbs from control mice and from I5 hAPPwt transgenic mice immunostained with anti-MOR28 reveal targeting to a single glomerulus ( P >0.50, two-tailed Student's t -test; n =8 (controls); n =9 (I5)). Scale bar=100 μm. Data presented as means±s.e.m. Full size image Selective expression of hAPPsw in OSNs alters connectivity To determine whether expression of hAPPsw exclusively in OSNs was sufficient to cause OSN axon mistargeting, we generated transgenic mouse lines that coexpress hAPPsw and the axonal marker human placental alkaline phosphatase (PLAP) in a conditional manner using the tetracycline transcriptional activator (TTA)/ TetO system [24] . These transgenic lines were crossed with a mouse line wherein the olfactory marker protein ( OMP ) gene was modified to co-express TTA ( Fig. 3a ) [25] . Immunohistochemical analysis of the olfactory epithelium of compound heterozygote mice demonstrated that a subset of the OSNs express hAPPsw ( Fig. 3b,c ). Immunostaining of the olfactory bulb indicated that OSNs expressing PLAP project broadly to the glomeruli of the olfactory bulb ( Fig. 3d,e ). Overall, approximately 12% (319/2653) of OSNs expressed the transgene products hAPPsw and PLAP, except in the very lateral region where the expression was markedly reduced, 1.4% (28/2017). The proportion of expression in the M71-defined subpopulation was 18.4% (28 hAPP+/152 OSNs), but the expression of hAPPsw in the lateral OSNs-expressing MOR28 was 0.19% (5 hAPP+/2604 OSNs). Importantly, we do not observe a shift in the pattern of expression of ORs over the olfactory epithelium. This mouse line expressing hAPPsw and PLAP was termed CORMAP ( C onditional, O lfactory Sensory Neuron- R estricted M osaic expression of A PPsw and P LAP). 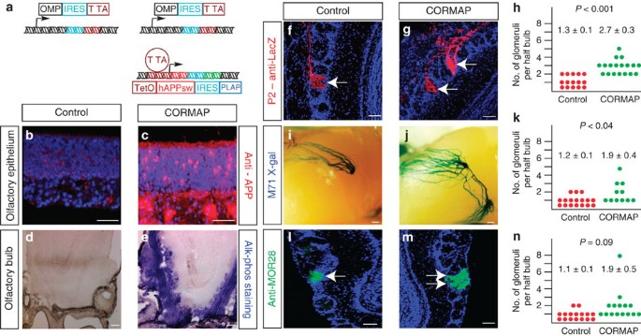Figure 3: Characterization of CORMAP mice. (a) Schematic diagram of the olfactory marker protein (OMP) gene locus altered by homologous recombination to introduce the internal ribosomal entry sequence (IRES) and tetracycline transcriptional activator (TTA; OMP-ivt) and the transgene encoding the operator sequenceTetOfollowed by hAPPsw, IRES and PLAP. (b,c) Coronal section of the medial olfactory epithelium from a control and a CORMAP mouse immunostained with an anti-APP antibody reveals background expression of the endogenous mouse APP in OSNs and ~12% of OSNs overexpress hAPPsw, respectively. (d,e) Coronal section of the olfactory bulb of a control and a CORMAP mouse colorimetrically stained for PLAP activity reveals that PLAP-labelled fibres target glomeruli in a stochastic pattern. (f–h) Representative images and quantification of olfactory bulbs from P2-ires-tauLacZ (tau-β-galactosidase fusion protein)/OMP-ivt and P2-ires-tauLacZ/CORMAP mice reveal targeting of LacZ-bearing neurons to one glomerulus (arrow) in control mice and targeting of LacZ-bearing axons to multiple glomeruli (arrows) in CORMAP mice (arrows identify glomeruli revealing P2-expressing fibres;P<0.001, two-tailed Student'st-test;n=15 (controls);n=18 (CORMAP)). (i–k) Representative images and quantification of olfactory bulbs from M71-ires-tauLacZ/OMP-ivt and littermate M71-ires-tauLacZ/CORMAP mice reveal targeting of LacZ-bearing neurons to one glomerulus in controls and to multiple glomeruli in CORMAP mice, with some fibres crossing between the lateral and medial projection loci. (P<0.04, two-tailed Student'st-test;n=17 (controls);n=11 (CORMAP)). (l–n) Representative images and quantification of olfactory bulbs from control and littermate CORMAP mice stained with anti-MOR28 antibody reveals MOR28-bearing axons targeting predominantly to a single glomerulus per half bulb in both lines (P<0.09, two-tailed Student'st-test;n=16 (controls);n=15 (CORMAP)). Scale bars=100 μm, except for (d,e) and (i,j) where scale bar=200 μm. Data presented as means±s.e.m. Figure 3: Characterization of CORMAP mice. ( a ) Schematic diagram of the olfactory marker protein ( OMP ) gene locus altered by homologous recombination to introduce the internal ribosomal entry sequence (IRES) and tetracycline transcriptional activator (TTA; OMP-ivt) and the transgene encoding the operator sequence TetO followed by hAPPsw, IRES and PLAP. ( b,c ) Coronal section of the medial olfactory epithelium from a control and a CORMAP mouse immunostained with an anti-APP antibody reveals background expression of the endogenous mouse APP in OSNs and ~12% of OSNs overexpress hAPPsw, respectively. ( d,e ) Coronal section of the olfactory bulb of a control and a CORMAP mouse colorimetrically stained for PLAP activity reveals that PLAP-labelled fibres target glomeruli in a stochastic pattern. ( f–h ) Representative images and quantification of olfactory bulbs from P2-ires-tauLacZ (tau-β-galactosidase fusion protein)/OMP-ivt and P2-ires-tauLacZ/CORMAP mice reveal targeting of LacZ-bearing neurons to one glomerulus (arrow) in control mice and targeting of LacZ-bearing axons to multiple glomeruli (arrows) in CORMAP mice (arrows identify glomeruli revealing P2-expressing fibres; P <0.001, two-tailed Student's t -test; n =15 (controls); n =18 (CORMAP)). ( i–k ) Representative images and quantification of olfactory bulbs from M71-ires-tauLacZ/OMP-ivt and littermate M71-ires-tauLacZ/CORMAP mice reveal targeting of LacZ-bearing neurons to one glomerulus in controls and to multiple glomeruli in CORMAP mice, with some fibres crossing between the lateral and medial projection loci. ( P <0.04, two-tailed Student's t -test; n =17 (controls); n =11 (CORMAP)). ( l–n ) Representative images and quantification of olfactory bulbs from control and littermate CORMAP mice stained with anti-MOR28 antibody reveals MOR28-bearing axons targeting predominantly to a single glomerulus per half bulb in both lines ( P <0.09, two-tailed Student's t -test; n =16 (controls); n =15 (CORMAP)). Scale bars=100 μm, except for ( d,e ) and ( i,j ) where scale bar=200 μm. Data presented as means±s.e.m. Full size image Immunostaining of CORMAP mice bearing a modified P2 gene, also expressing the tau-LacZ fusion protein [20] , revealed multiple glomeruli receiving fibres labelled with LacZ, which was significantly different from immunostaining littermate P2/tau-LacZ mice expressing only the TTA transcription factor alone ( Fig. 3f–h ; P <0.001; two-tailed Student's t -test; n =15 (control); n =18 (CORMAP)). Similarly, crossing CORMAP mice with a mouse line with a modified M71 gene, also expressing the tau-LacZ fusion protein [26] , revealed multiple glomeruli receiving LacZ fibres per half bulb ( Fig. 3i–k ; P <0.04; two-tailed Student's t -test; n =17 (control); n =12 (CORMAP)). OSNs-expressing MOR28 predominantly targeted one glomerulus per half bulb in CORMAP mice and control littermates ( Fig. 3l–n ); the intact targeting likely reflects the scant transgene expression in that region of the epithelium. Overall, the axon guidance phenotypes were similar to those observed in Tg2576, indicating that restricted expression of hAPPsw to OSNs is sufficient to disrupt their axon targeting. Selective expression of hAPPmv in OSNs maintains connectivity As hAPPsw facilitates production of Aβ, we generated transgenic mouse lines that coexpresses hAPPmv ( Fig. 1b ), a hAPP isoform that impairs Aβ production [12] , and the axonal marker mCherry in a conditional manner as described above ( Fig. 4a ). Similarly, a subset of medial OSNs (17.6%; 239/1366) expressed hAPPmv and mCherry ( Fig. 4b,c ), and smaller subset of lateral OSNs (4.7%; 37/782) expressed the transgene. OSNs expressing mCherry projected broadly to the glomeruli in the olfactory bulb ( Fig. 4d,e ). The proportion of transgene expression in the MOR28-defined subpopulation mirrored the ambient density of the lateral epithelium (4.6%; 26 hAPP+/568 OSNs). Moreover, we did not observe a shift in the pattern of expression of ORs over the olfactory epithelium. This mouse line expressing hAPPmv and mcherry was termed CORMAC ( C onditional, O lfactory Sensory Neuron- R estricted M osaic expression of A PPmv and m C herry). The number of glomeruli targeted by OSNs coexpressing P2 and tau-LacZ in CORMAC mice was similar to control littermates ( Fig. 4f–h ). Similarly, the distribution of targeted glomeruli by M71-expressing OSNs did not differ between CORMAC mice and control littermates ( Fig. 4i–k ). Moreover, predominantly one glomerulus per half bulb was labelled with an antibody against MOR28 in both hAPPmv and control littermates ( Fig. 4l–n ). In summary, the patterns of connectivity of OSNs in CORMAC mice were preserved, thus demonstrating the specificity of the hAPPsw phenotype. 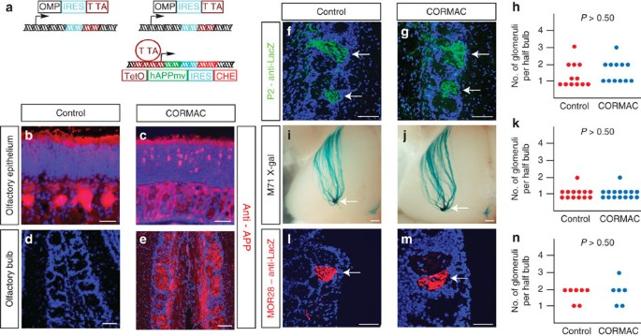Figure 4: Characterization of CORMAC mice. (a) Schematic diagram of theOMPgene locus altered by homologous recombination to introduce the IRES and TTA(OMP-ivt) and the transgene encoding the operator sequenceTetOfollowed by hAPPmv (hAPP M671V), IRES and the mCherry (CHE). (b,c) Coronal section of the medial olfactory epithelium from control and CORMAC mice immunostained with an anti-APP antibody reveals background expression of the endogenous mouse APP in OSNs and ~18% of OSNs overexpressing hAPPmv, respectively. (d,e) Coronal sections of olfactory bulbs from a control mouse and a CORMAC mouse reveal fibres containing mCherry target glomeruli in a stochastic pattern. (f–h) Representative images and quantification of olfactory bulbs from P2-ires-tauLacZ/OMP-ivt and P2-ires-tauLacZ/CORMAC mice reveal targeting of LacZ-bearing neurons to equal glomeruli (arrows) in both control and CORMAC mice. (P>0.50, two-tailed Student'st-test;n=12 (controls);n=12 (CORMAC)). (i–k) Representative images and quantification of olfactory bulbs from M71-ires-tauLacZ/OMP-ivt and littermate M71-ires-tauLacZ/CORMAC mice reveal targeting of LacZ-bearing neurons to one glomerulus in both control and CORMAC mice. (P>0.50, two-tailed Student'st-test;n=13 (controls);n=15 (CORMAC)). (l–n) Representative images and quantification of olfactory bulbs from MOR28-ires-tauLacZ/OMP-ivt and littermate MOR28-ires-tauLacZ/CORMAC mice reveal targeting of LacZ-bearing neurons to one glomerulus (arrow) in both control and CORMAC mice (P>0.50, two-tailed Student'st-test;n=7 (controls);n=6 (CORMAC)). Scale bars=100 μm, except for (i,j) where scale bar=200 μm. Figure 4: Characterization of CORMAC mice. ( a ) Schematic diagram of the OMP gene locus altered by homologous recombination to introduce the IRES and TTA(OMP-ivt) and the transgene encoding the operator sequence TetO followed by hAPPmv (hAPP M671V), IRES and the mCherry (CHE). ( b,c ) Coronal section of the medial olfactory epithelium from control and CORMAC mice immunostained with an anti-APP antibody reveals background expression of the endogenous mouse APP in OSNs and ~18% of OSNs overexpressing hAPPmv, respectively. ( d,e ) Coronal sections of olfactory bulbs from a control mouse and a CORMAC mouse reveal fibres containing mCherry target glomeruli in a stochastic pattern. ( f–h ) Representative images and quantification of olfactory bulbs from P2-ires-tauLacZ/OMP-ivt and P2-ires-tauLacZ/CORMAC mice reveal targeting of LacZ-bearing neurons to equal glomeruli (arrows) in both control and CORMAC mice. ( P >0.50, two-tailed Student's t -test; n =12 (controls); n =12 (CORMAC)). ( i–k ) Representative images and quantification of olfactory bulbs from M71-ires-tauLacZ/OMP-ivt and littermate M71-ires-tauLacZ/CORMAC mice reveal targeting of LacZ-bearing neurons to one glomerulus in both control and CORMAC mice. ( P >0.50, two-tailed Student's t -test; n =13 (controls); n =15 (CORMAC)). ( l–n ) Representative images and quantification of olfactory bulbs from MOR28-ires-tauLacZ/OMP-ivt and littermate MOR28-ires-tauLacZ/CORMAC mice reveal targeting of LacZ-bearing neurons to one glomerulus (arrow) in both control and CORMAC mice ( P >0.50, two-tailed Student's t -test; n =7 (controls); n =6 (CORMAC)). Scale bars=100 μm, except for ( i,j ) where scale bar=200 μm. Full size image A mouse line overexpressing a synthetic APP isoform (mouse/human chimeric protein with Swedish and Indiana mutations) was recently reported to generate high levels of human Aβ, which in turn caused accelerated OSN death [27] . In our study, levels of activated caspase-3 and the density of OSN subpopulations in Tg2576, CORMAP or CORMAC lines were not significantly different from control littermates ( Supplementary Fig. S2 ). Olfactory deficits correlate with altered connectivity The OSN-specific restricted expression of hAPP isoforms in both CORMAP and CORMAC lines affords the opportunity to determine the functional consequence of these connectivity deficits using odour-evoked behavioural assays without the potential confounds that central neural circuits may be affected by hAPP expression. We assessed olfactory function in these lines using two paradigms. The response to 2,3,5-trimethyl-3-thiazoline (TMT), an odourant isolated from fox faeces with an innate aversive response to mice, was monitored ( Fig. 5a ) [28] . CORMAP, but not CORMAC, mice spent significantly more time within region of the arena where TMT was present ( Fig. 5b,c ). Moreover, in an olfactory assay monitoring appetitive behaviour [29] , food-restricted CORMAP mice took significantly more time to find food buried under mouse bedding relative to littermate controls ( Fig. 5d,e ). Together, these olfactory assays indicate that compromised olfactory function correlates with alterations in structural connectivity of the peripheral olfactory neural circuit. 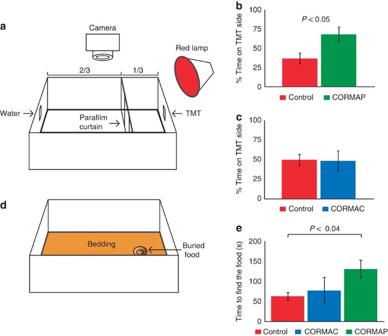Figure 5: Olfactory behavioural deficit in the CORMAP mice but not in CORMAC mice. (a) Schematic representation of the behavioural arena to assess the response to 2,3,5-trimethyl-3-thiazoline (TMT), an odour isolated from fox faeces that triggers an innate aversion response in mice. (b,c) Percentage of time that each mouse spent in a compartment with the innately aversive odour TMT relative to a compartment with water for a 3-min period. Relative to littermate controls, CORMAC (hAPPmv) but not CORMAP (hAPPsw) mice avoided TMT. (P<0.05; one-way analysis of variance (ANOVA);n=5 pairs of littermate mice for each genotype with ages ranging from 3 to 5 months). (d) Schematic representation of the behavioural arena to find the buried food. (e) Graphical representation of time to find food for controls, CORMAC and CORMAP mice. Relative to controls, CORMAP but not CORMAC required a significantly longer time to find the food (P<0.04; one-way ANOVA;n=4 (control), three (CORMAC) and four (CORMAP) with ages ranging from 3 to 6 months). Error bars=s.e.m. Figure 5: Olfactory behavioural deficit in the CORMAP mice but not in CORMAC mice. ( a ) Schematic representation of the behavioural arena to assess the response to 2,3,5-trimethyl-3-thiazoline (TMT), an odour isolated from fox faeces that triggers an innate aversion response in mice. ( b,c ) Percentage of time that each mouse spent in a compartment with the innately aversive odour TMT relative to a compartment with water for a 3-min period. Relative to littermate controls, CORMAC (hAPPmv) but not CORMAP (hAPPsw) mice avoided TMT. ( P <0.05; one-way analysis of variance (ANOVA); n =5 pairs of littermate mice for each genotype with ages ranging from 3 to 5 months). ( d ) Schematic representation of the behavioural arena to find the buried food. ( e ) Graphical representation of time to find food for controls, CORMAC and CORMAP mice. Relative to controls, CORMAP but not CORMAC required a significantly longer time to find the food ( P <0.04; one-way ANOVA; n =4 (control), three (CORMAC) and four (CORMAP) with ages ranging from 3 to 6 months). Error bars=s.e.m. Full size image Reduced expression of activity-dependent gene products To confirm that the functional responses of OSNs was compromised in the CORMAP line, we quantified tyrosine hydroxylase (TH) expression by periglomerular dopaminergic neurons as a surrogate marker of OSN input activity [30] . Statistically significant reductions in levels of the TH signal were measured in the glomerular layer of CORMAP mice relative to wild-type littermates ( Fig. 6a–c ; P <0.01; two-tailed Student's t -test; n =5 mice per genotype) that had been housed in the same cage. In addition, we quantified the expression of the immediate early gene Arc in periglomerular and tufted neurons of CORMAP mice relative to littermate controls. We observe a significant reduction in the number of neurons expressing Arc ( Fig. 6d-f ; P <0.01; two-tailed Student's t -test; n =60–100 per genotype). As periglomerular and tufted neurons in the olfactory bulbs of CORMAP mice do not express hAPPsw, we interpret these reduced levels of TH and Arc as reflecting reduced input from OSNs. 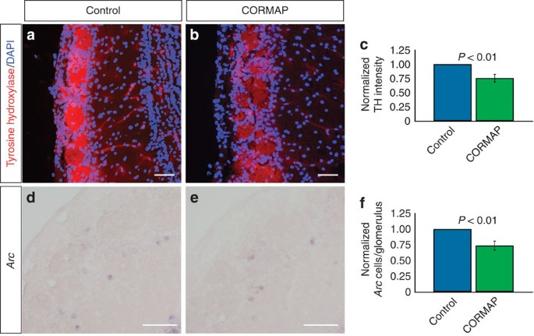Figure 6: Reduced induction of OSN activity-dependent genes in CORMAP mice olfactory bulbs. (a) Representative image of olfactory bulbs from a control mouse immunostained with an antibody recognizing tyrosine hydroxylase (TH; red) and a nuclear stain (blue). (b) Representative image of olfactory bulbs from a CORMAP mouse immunostained with an antibody recognizing TH (red) and a nuclear stain (blue). (c) Quantification of the intensity of TH staining in glomeruli of CORMAP (n=5 bulbs) and littermate control mice (n=5 bulbs) reveals a statistically significant difference (P<0.01; two-tailed Student'st-test). (d) Representative image of an olfactory bulb from a control mouse followingin situhybridization with an antisenseArcprobe. (e) Representative image of an olfactory bulb from a CORMAP mouse followingin situhybridization with an antisenseArcprobe. (f) Quantification of number of periglomerular and tufted neurons expressingArcin matched regions of the olfactory bulbs from CORMAP (n=5) and littermate control mice (n=5) reveals a significant difference (P<0.01; two-tailed Student'st-test;n=60–100 per genotype). Scale bar=100 μm. Error bars=s.e.m. Figure 6: Reduced induction of OSN activity-dependent genes in CORMAP mice olfactory bulbs. ( a ) Representative image of olfactory bulbs from a control mouse immunostained with an antibody recognizing tyrosine hydroxylase (TH; red) and a nuclear stain (blue). ( b ) Representative image of olfactory bulbs from a CORMAP mouse immunostained with an antibody recognizing TH (red) and a nuclear stain (blue). ( c ) Quantification of the intensity of TH staining in glomeruli of CORMAP ( n =5 bulbs) and littermate control mice ( n =5 bulbs) reveals a statistically significant difference ( P <0.01; two-tailed Student's t -test). ( d ) Representative image of an olfactory bulb from a control mouse following in situ hybridization with an antisense Arc probe. ( e ) Representative image of an olfactory bulb from a CORMAP mouse following in situ hybridization with an antisense Arc probe. ( f ) Quantification of number of periglomerular and tufted neurons expressing Arc in matched regions of the olfactory bulbs from CORMAP ( n =5) and littermate control mice ( n =5) reveals a significant difference ( P <0.01; two-tailed Student's t -test; n =60–100 per genotype). Scale bar=100 μm. Error bars=s.e.m. Full size image Expression Aβ40 or Aβ42 disturbs OSN axon targeting The specificity of the hAPPsw phenotype implies that a beta-site APP cleaving enzyme 1 (BACE1) cleavage product of APP mediates axon dysfunction of OSNs. To determine whether the expression of human Aβ disrupts axon targeting of OSNs, we transduced the olfactory epithelia of mice with adeno-associated virus (AAV) expressing either the Bri-Aβ40 fusion protein or the Bri-Aβ42 fusion protein, which are cleaved sequentially by furin to secrete the human Aβ40 or Aβ42 peptide, respectively [31] . We instilled one naris of M71/tau-LacZ mice with AAV8 expressing either Bri-Aβ40 or Bri-Aβ42. The uninfected side served as a control. After 12 weeks, examination of M71-expressing OSNs revealed disturbed axon targeting on the infected side compared with the non-infected side ( Fig. 7a–c ). In control experiments, infection of AAV8 expressing GFP in one naris did not disturb M71 axon targeting (data not shown). Immunostaining of the olfactory epithelia from infected mice using the anti-hAPP and Aβ antibody 6E10 revealed expression in the superficial layers of the olfactory epithelium. The cells expressing human Aβ40 co-stained with a marker for non-neuronal sustentacular cells ( Supplementary Fig. S3a–d ). Similarly, the infected side with Bri-Aβ42-expressing virus also caused axon mistargeting of M71-expressing axons ( Fig. 7d–f ). Of note, immunostaining of both the infected olfactory epithelium and the ipsilateral olfactory bulb with 6E10 did not reveal evidence of amyloid deposition ( Supplementary Fig. S3e ); moreover, formic acid extraction of the olfactory bulbs from the Bri-Aβ42-infected mice followed by enzyme-linked immunosorbent assay did not detect Aβ42 (data not shown). These data support an extracellular mechanism of action of Aβ (that is likely to be soluble) to disturb axon targeting of OSNs. We cannot exclude the possibility that other cleavage products of APP contribute to the hAPPsw phenotype. 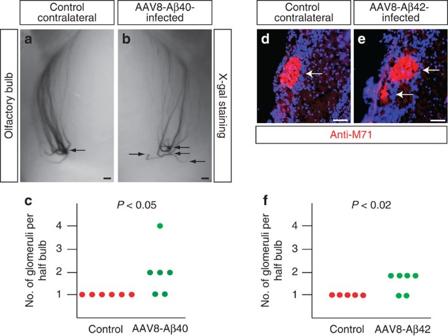Figure 7: Aβ40 and Aβ42expression in the olfactory epithelium alters OSN axon targeting. (a,b) Representative images of the olfactory bulbs from an M71-ires-tauLacZ mouse infected with AAV8-BriAβ40 that were stained with X-gal (arrows indicate glomeruli receiving M71-expressing fibres). Scale bar=200 μm. (c) Quantification of number of glomeruli receiving M71-expressing axons revealed a significant degree of mistargeting in the olfactory bulb ipsilateral to the AAV8-BriAβ40 infection (P<0.05; two-tailed Student'st-test;n=6 per genotype). (d,e) Representative images of the olfactory bulbs from a mouse infected with AAV8-BriAβ42 immunostained with antibody that recognizes M71 (arrows identify glomeruli revealing M71-expressing fibres). Scale bar=100 μm. (f) Quantification of number of glomeruli receiving M71-expressing axons revealed a significant degree of mistargeting in the olfactory bulb ipsilateral to the AAV8-BriAβ42 infection (P<0.02; two-tailed Student'st-test;n=5 (controls);n=6 (AAV8-BriAβ42). Figure 7: Aβ40 and Aβ42expression in the olfactory epithelium alters OSN axon targeting. ( a , b ) Representative images of the olfactory bulbs from an M71-ires-tauLacZ mouse infected with AAV8-BriAβ40 that were stained with X-gal (arrows indicate glomeruli receiving M71-expressing fibres). Scale bar=200 μm. ( c ) Quantification of number of glomeruli receiving M71-expressing axons revealed a significant degree of mistargeting in the olfactory bulb ipsilateral to the AAV8-BriAβ40 infection ( P <0.05; two-tailed Student's t -test; n =6 per genotype). ( d,e ) Representative images of the olfactory bulbs from a mouse infected with AAV8-BriAβ42 immunostained with antibody that recognizes M71 (arrows identify glomeruli revealing M71-expressing fibres). Scale bar=100 μm. ( f ) Quantification of number of glomeruli receiving M71-expressing axons revealed a significant degree of mistargeting in the olfactory bulb ipsilateral to the AAV8-BriAβ42 infection ( P <0.02; two-tailed Student's t -test; n =5 (controls); n =6 (AAV8-BriAβ42). Full size image The increasing awareness of the susceptibility of olfactory acuity in people with prodromal neurodegenerative disease, relative to other sensory modalities, and our deeper understanding of the physiology underlying olfactory perception [32] , [33] have made the olfactory neural network in animals a more widely used model to investigate mechanisms of neurodegenerative disease [34] , [35] . The amenability of the mouse peripheral olfactory neural circuit to genetic, imaging and behavioural characterization renders it a powerful model system to elucidate the actions of disease proteins [16] , [27] . One of the unique aspects of this neural circuit is the continuous renewal of OSNs in adults [36] , necessitating precise axon targeting throughout its lifetime to maintain the integrity of the circuit. We exploit this physiologic structural plasticity to visualize dysfunction caused by the expression of genes that cause neurological disease. Here, we report that expression of the Swedish mutation of hAPP in mice in vivo alters the connectivity and function of the peripheral olfactory neural circuit in the absence of plaques. Our initial observation of this axon guidance phenotype occurred in well-characterized lines that overexpress hAPPsw throughout the brain. Taking advantage of methodology to specifically express genes in the peripheral olfactory neural circuit [37] , we generated and examined two lines of mice that overexpress hAPP alleles exclusively in the presynaptic neurons of this circuit. Aβ production is facilitated in one line that expresses hAPPsw and impeded in the other line that expresses hAPPmv [12] . Overproduction of hAPPsw in the presynaptic neurons was sufficient to perturb the structural connectivity of the peripheral olfactory neural circuit. The absence of a phenotype in the hAPPmv line corroborated our findings in the mouse line overexpressing the wild-type form of hAPP. Together with preserved fidelity of axon targeting in the I5 line overexpressing wild-type hAPP throughout the brain, these important controls indicate that overexpression of hAPP is not sufficient to alter OSN axonal connectivity. Rather, our findings suggest that products of BACE1-mediated cleavage of APP critically modulate neuronal function—in congruence with results from studies in hippocampal slices [13] , [15] , [38] , in induced human neurons derived from skin fibroblasts [39] and studies of BACE1 heterozygous and null mice [40] . We postulate that Aβ is the BACE1 cleavage product of APP involved in mediating the connectivity phenotype. The presence of the connectivity phenotype in mice expressing hAPPsw, but not in the I5 line expressing hAPPwt and the CORMAC line expressing hAPPmv, supports this hypothesis. Moreover, expression of human Aβ40 or human Aβ42 in the olfactory epithelium using a viral vector delivered intranasally phenocopies the alteration in the projection map of OSN axons. As we observe these axon targeting deficits in young mice before the onset of plaques in the broadly expressing lines and as we do not observe amyloid plaques in lines that overexpress hAPP isoforms exclusively in OSNs or in the virally infected mice, this novel axonal phenotype is independent of amyloid plaque deposition. This phenotype is unlikely to be caused by an in utero anomaly, as we can induce it in adult control mice by intranasal expression of Aβ40 or Aβ42. Together, these data are consistent with a model that soluble Aβ triggers axonal dysfunction in the absence of amyloid plaques in vivo , although we cannot disprove that insoluble Aβ could also cause similar changes. In addition to altering structural connectivity, expression of hAPPsw exclusively in OSNs has functional consequences as indicated by two lines of evidence. First, relative to control littermates or CORMAC mice, CORMAP mice exhibit significant reductions in olfactory acuity in two distinct behavioural paradigms, one paradigm employing an odour that evokes an aversive response while the other paradigm employs an odour that evokes an appetitive response. We interpret these olfactory-mediated behavioural responses as reflecting the function of the peripheral olfactory neural circuit in CORMAP and CORMAC lines—an interpretation afforded by the restricted expression pattern of hAPPsw and hAPPmv, respectively. Deficits in an odour habituation paradigm have been reported in Tg2576 mice at ages 6–7 months that correlated with amyloid plaque deposition [34] . By contrast, the behavioural phenotype of CORMAP mice is detectable at 3–5 months of age and is independent of amyloid plaques. Second, the expression of two independent activity-dependent markers in postsynaptic neurons in the olfactory bulb were significantly reduced in CORMAP mice relative to littermate controls. The magnitude of reduction of these activity-dependent markers (~25%) exceeds the frequency of expression of hAPPsw in mature OSNs (~12%). This disproportional response in the functional data raises the possibility that hAPPsw may be acting in a non-cell autonomous manner, as seen in studies in hippocampal slices by Malinow's laboratory [13] , [38] . Our attempts to determine whether a non-cell autonomous mechanism underlies the structural connectivity phenotype in the CORMAP line have not been conclusive to date. Future studies employing expression of hAPP isoforms by specific OR promotors are aimed to address this question directly. Our data illustrate a detrimental effect of heightened Aβ levels on a neural circuit in the absence of plaques. The CORMAP line offers a quantifiable outcome of the actions of hAPPsw, and likely Aβ, which is distinct from amyloid plaque production and that could be utilized to assess therapies targeting aberrant neural plasticity due to Aβ. Although olfactory deficits have been shown in patients with prodromal and mild AD, demonstration of alterations in the map of OSN projections in the human olfactory bulb in AD is necessary to postulate that the CORMAP mouse is a model for the disease. Increasing evidence indicates that Aβ levels rise after neuronal injury by increased expression of APP and/or BACE1 [41] . Established risk factors for late-onset AD, for example, head trauma and vascular insults, result in elevated Aβ production [42] . Further delineation of the mechanism of action of human Aβ in this model system may provide insight into neural circuit and network dysfunction in the long, preclinical stage of AD. Animals All experiments were in accordance with protocols approved by the Institutional Animal Care and Use Committee of Massachusetts General Hospital. Tg2576 mice overexpressing hAPPsw [22] were obtained from Taconic Farms (Hudson, NY, USA). I5 hAPPwt mice [9] and M71-ires-tauLacZ were obtained from Jackson Labs (Bar Harbor, ME, USA). P2-ires-GFP [20] and P2-ires-tauLacZ [43] mice were a gift from Richard Axel. Generation and characterization of CORMAP and CORMAC mice Transgenic constructs were generated using the hAPPsw695 cDNA, ires-PLAP [44] and pBSRV [37] , which contained the tetO sequence followed by an artificial intron and splice site, the Pac site and an SV40 polyadenylation signal. For the CORMAC mice, the hAPPsw695 (K670N; M671L) cDNA was mutated to the mv genotype (M671V) by PCR mutagenesis (Stratagene) and confirmed by sequencing. A DNA fragment encoding ires-mcherry was isolated and the hAPPmv–ires-mcherry fragment was cloned and injected. The founder mouse was crossed with OMP-ires-tTA mice [25] . Compound heterozygote mice of the founders for the CORMAP line expressed hAPPsw and PLAP in ~12% of OSNs and not elsewhere in the brain. This line was backcrossed into C57/BL6 for six generations. Compound heterozygote mice of a founder for the CORMAC line expressed hAPPsw and mCherry in approximately 18% of OSNs and not elsewhere in the brain. This line was backcrossed into C57/BL6 for six generations. The ages of mice used in this study ranged from 3 weeks to 1 year. Immunohistochemistry Standard procedures were used as previously described [45] . The mice were anaesthetized with an intraperitoneal injection of 3,3,3-tribromoethanol (1.25% in PBS 30 μl g −1 body weight). Following thoracotomy, intracardiac perfusion with 10 ml of PBS (pH 7.4) was performed. For anti-GFP and anti-LacZ immunostaining, the mice were subsequently perfused with 2% paraformaldehyde in PBS (pH 7.4). The olfactory turbinates and olfactory bulbs were dissected intact, incubated in 30% sucrose in PBS at 4 °C overnight and embedded in optical coherence tomography (Sakura) or M1 (Shandon) in a dry ice/ethanol bath. Twenty micrometre coronal sections were cut on a cryostat (Microm) and collected on SuperFrost slides (Fisher). For immunostaining using the MOR28 and M71 antibodies, the sections were post-fixed with 1% paraformaldehyde in PBS for 8 min at room temperature. All sections were washed three times in PBS for 10 min, permeabilized in 0.1% Triton X-100 in PBS (PT) for 30 min at room temperature, blocked in 5% heat-inactivated horse serum in PT (PTS) for 1 h at room temperature, incubated with primary antibody in PTS under a Hybrislip (Invitrogen) overnight in a humidified chamber at 4 °C, washed three times with PT for 10 min, blocked with PTS for 30 min at room temperature, incubated with a fluorescent-conjugated secondary antibody in PTS with DAPI (Invitrogen, 1/1000) for 2 h at room temperature, washed briefly in PBS, and Vectashield was applied to each slide and coverslipped. Slides were analysed using a Zeiss LSM-510 confocal microscope or a Leica confocal microscope and analysed using ImageJ (NIH). Primary antibodies included rabbit anti-GFP (Molecular Probes; 1/1000); sheep anti-GFP (Biogenesis; 1/1000); rabbit anti-LacZ (Cappel; 1/1000); rabbit anti-APP (6900; Zymed; 1/1000); mouse anti-hAPP and Aβ (4G8 and 6E10, Covance; 1/1000); rabbit anti-MOR28 (1/3000) [23] , guinea pig anti-M71 (1/1000) [23] , rabbit anti-activated caspase 3 (Cell Signaling; 1/500); rabbit anti-TROMA (Molecular Probes; 1:10) and mouse anti-tyrosine hydroxylase (Millipore; 1/500). Secondary antibodies were Alexa 488-conjugated donkey anti-rabbit Ig (Molecular Probes; 1/500), Alexa 488-conjugated donkey anti-sheep Ig (Molecular Probes; 1/500), Cy3-conjugated donkey anti-guinea pig Ig (Jackson Immunoresearch; 1/500), Cy3-conjugated rat anti-mouse Ig (Jackson Immunoresearch; 1/500). In situ hybridization Twenty-micrometre-thick, fresh frozen tissue sections were placed on Superfrost slides (Fisher Scientific). The sections were dried for 45 min at room temperature before fixing with 4% paraformaldehyde for 15 min, and washed three times in 1×DEPC (diethylpyrocarbonate)-treated PBS containing 1 mM MgCl 2 . Slides were then immersed in a solution containing 270 ml of DEPC-treated water, 30 ml of 1 M triethanolamine and 750 μl of 95% acetic anhydride for 10 min, and subsequently washed three times in 1×DEPC-treated PBS containing 1 mM MgCl 2 . Slides were then blocked for 2 h with hybridization buffer: 0.1% Tween20, 50% formamide, 5×SSC, 5×Denhardts, 5 mM EDTA, 10 mM NaH2PO4 at pH. 8.0, 50 mM Tris pH 8.0, 250 μg ml −1 salmon sperm DNA, 100 μg ml −1 tRNA and 100 μg ml −1 yeast RNA. Slides were dabbed dry and Arc antisense RNA probes [46] (100 μg ml −1 ), preheated for 5 min at 80 °C and cooled on ice for 2 min, were applied to the slides and sealed in a humidified chamber at 65 °C overnight. After 18 h, the slides were washed at 65 °C three times with 5×SSC for 15 min, and then three times with 0.2×SSC for 20 min. After blocking in 1× in situ hybridization blocking solution (Roche) for 1 h, slides were dabbed dry and a sheep antibody-recognizing digoxetin (1/3000, Roche) was applied overnight. The next day, the RNA probe was detected using the HNPP fluorescent detection kit (Roche) or BCIP/NBT (Promega). Whole mount Whole mount analyses were performed as previously described [47] . Briefly, mice harbouring the P2-ires-GFP allele were anaesthesized as described above. The skull was dissected and then divided sagittally, and the dura was removed from the medial surface of each olfactory bulb. Each whole mount was placed in PBS with 2 mM MgCl 2 and then imaged using a Leica confocal imaging system. Preparation and staining of olfactory bulbs expressing tau-LacZ was performed as previously described [20] . AAV infection AAV was introduced intranasally in one naris of a 2-month-old M71-ires-tauLacZ mice (Bri-Aβ40) or control mice (Bri-Aβ42) by diluting 2.5 μl of AAV8 virus with 57.5 μl of 2% methylcellulose in PBS (1% final concentration; 5×10 12 pfu) as previously described [48] . Analysis by immunohistochemistry and whole mount preparation occurred 90 days after infection. Behaviour The TMT assay was derived from the curtain assay [28] . Briefly, the experiment was performed in the dark during the nocturnal phase of the day. The behavioural arena ( Fig. 4a ) was placed in a chemical hood. Mice (age range 3–5 months) were habituated to the arena three times for 10 min with blank filter papers. After 7 min of the third habituation, the filter papers were swapped with identical filter papers with 20 μl of water or TMT, respectively. The remaining 3 min were video-recorded and scored in a blinded fashion. One-way analysis of variance and unpaired Student's t -tests were used to analyse the data. The hidden food assay was derived from similar assays previously described [29] , [49] . The mice (age 3–9 months) were food-restricted for 24 h and then habituated in an 82×63×18 cm arena with 2 cm autoclaved mouse bedding for 5 min. Then they are returned to their home cage for 30 min. Each animal was placed back in the arena with fresh autoclaved bedding covering 1 g of ground food pellet placed in one specific location. The trial was analysed in real time using a stopwatch until the food was ingested. The experimenters recording the latency to eat the food were blinded to the genotype. The results between the two experimenters were not significantly different. Each animal was tested once. Statistical analysis One-way analysis of variance and unpaired Student's t -tests were performed using SAS, Microsoft Excel or Apple Numbers, and results are presented as mean±s.e.m. How to cite this article: Cao, L. et al . Aβ alters the connectivity of olfactory neurons in the absence of amyloid plaques in vivo . Nat. Commun. 3:1009 doi: 10.1038/ncomms2013 (2012).